Mapping multiple photonic qubits into and out of one solid-state atomic ensemble The future challenge of quantum communication is scalable quantum networks, which require coherent and reversible mapping of photonic qubits onto atomic systems (quantum memories). A crucial requirement for realistic networks is the ability to efficiently store multiple qubits in one quantum memory. In this study, we show a coherent and reversible mapping of 64 optical modes at the single-photon level in the time domain onto one solid-state ensemble of rare-earth ions. Our light–matter interface is based on a high-bandwidth (100 MHz) atomic frequency comb, with a predetermined storage time of ≳ 1 μs. We can then encode many qubits in short (<10 ns) temporal modes (time-bin qubits). We show the good coherence of mapping by simultaneously storing and analysing multiple time-bin qubits. Quantum communication [1] offers the possibility of secure transmission of messages using quantum key distribution [2] and teleportation of unknown quantum states [3] . Quantum communication relies on the creation, manipulation and transmission of qubits in photonic channels. Photons have proven to be robust carriers of quantum information. Yet, the transmission of photons through a fibre link, for instance, is inherently a lossy process. This leads to a probabilistic nature of the outcome of experiments. In large-scale quantum networks [4] , the possibility of synchronizing independent and probabilistic quantum channels is required for scalability [5] , [6] . A quantum memory enables this by momentarily holding a photon and then releasing it when another part of the network is ready. To reach reasonable rates in a realistic network, it is necessary to use multiplexing [7] , which demands quantum memories capable of storing many single photons in different modes. A quantum memory requires a coherent medium with strong coupling to a light mode. Strong and coherent interactions can be found in ensembles of atoms [8] , for instance, alkali atoms or rare-earth (RE) ions doped into crystals. The latter are attractive for quantum storage applications, as they provide solid-state systems with a large number of stationary atoms having excellent coherence properties. Optical coherence times of up to milliseconds [9] and spin coherence times greater than seconds [10] have been shown at low temperature ( ≲ 4 K). A quantum memory also requires a scheme for achieving efficient and reversible mapping of the photonic qubit onto the atomic ensemble. Techniques investigated include stopped light based on electromagnetically induced transparency (EIT) [11] , [12] , [13] , Raman interactions [14] , [15] , [16] , [17] or photon-echo-based schemes [18] , [19] , [20] , [21] , [22] . Much progress has been made in terms of quantum memory efficiency [13] , [23] and storage time [24] , [25] . Storage of multiple qubits is challenging, however, because it necessitates a quantum memory that can store many optical modes into which qubits can be encoded. A mode can be defined in time, space or frequency. Lan et al . [26] recently showed that a multiplexed quantum memory can be achieved by storing several single excitations in separate spatial modes, each functioning as an independent memory. Time multiplexing, as used in classical communication, has the great advantage of requiring only a single spatial mode [7] , [21] , [27] , hence a single quantum memory. Moreover, each pair of temporal modes can be used to encode different time-bin qubits [1] , or more generally d modes can encode a qudit. Time-bin qubits are widely used in fibre-based quantum communication [1] , [2] because of their resilience against polarization decoherence in fibres. Temporal multimode storage is difficult, however, because of the scaling of the number of stored modes N m as a function of optical depth d of the storage medium [21] , [27] . For EIT and Raman interactions, N m scales as √ d , making it very difficult to store many modes [27] . Recently, we proposed [21] a multimode storage scheme based on atomic frequency combs (AFC) with a high intrinsic temporal multimode capacity [21] , [27] . Using this method, we recently showed [22] that a weak coherent state | α 〉 L with mean photon number n̄ =| α | 2 <1 can be coherently and reversibly mapped onto a YVO 4 crystal doped with neodymium ions. Later experiments [28] , [29] , [30] , [31] in other RE-doped materials have improved the overall storage efficiency (35%) and storage time (20 μs). Yet, in these experiments, only a maximum of four modes have actually been stored at the single-photon level; thus, the predicted [21] , [27] high multimode capacity has yet to be shown experimentally. In this study, we show reversible mapping of 64 temporal modes containing weak coherent states at the single-photon level onto one atomic ensemble in a single spatial mode using an AFC-based light–matter interface. The light–matter interface An AFC is based on a periodic modulation (with periodicity Δ) of the absorption profile of an inhomogeneously broadened optical transition | g 〉→| e 〉 (see Fig. 1 ). The modulation should ideally consist of sharp teeth (with full-width at half-maximum γ ) having a high peak absorption depth d (see Fig. 1b ). Such a modulation can be created by optical pumping techniques (see Experiment section and Methods). This requires an atomic ensemble with a static inhomogeneous broadening and many independently addressable spectral channels. This can be found in RE-doped solids in which inhomogeneous broadening is of the order of 1–10 GHz and the homogeneous linewidth is of the order of 1–100 kHz when cooled to <4 K. When a weak photonic coherent state | α 〉 L with n̄ <1 is absorbed by the atoms in the comb, the state of the atoms can be written as | α 〉 A =| G 〉+ α | W 〉+ O ( α 2 ). 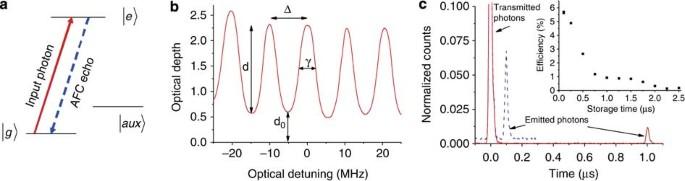Figure 1: AFC storage scheme. (a) Simplified level scheme of the Nd ions doped into Y2SiO5. We use the optical transition at 883 nm between the4I9/2ground state and4F3/2excited state. The former is split into two Zeeman levels by a 0.3 T magnetic field (|g〉 and |aux〉). The experiment is conducted on |g〉−|e〉, where the absorption profile is shaped into an AFC by optically pumping atoms into |aux〉. The basic idea is to send in a pulse sequence on |g〉−|e〉 that has a periodic spectral density (due its Fourier spectrum). Some of the excited atoms have a certain probability to spontaneously de-excite to |aux〉. The atoms left behind in |g〉 form the grating (see panel (b)). To build up a deep grating, the sequence is repeated many times (up to the timescale of the population relaxation between |g〉 and |aux〉). More details on the preparation can be found in the Experimental setup and Methods section. (b) An example of a generated comb with periodicity Δ=10 MHz. The relevant AFC parameters defined in the text are indicated. (c) Mapping of weak coherent states withn̄=0.5 (in a single temporal mode) onto the Nd-doped crystal. Shown are two different experiments with Δ=10 MHz (dashed line offset vertically) and 1 MHz (solid line). The photons that are transmitted without being absorbed are detected att=0, whereas the absorbed and reemitted photons are detected aroundt=1/Δ. The vertical scale has been normalized such that it yields efficiency. Inset: The overall write and read efficiency as a function of 1/Δ. Here, | G 〉=| g 1… g N 〉 represents the ground atomic state and Figure 1: AFC storage scheme. ( a ) Simplified level scheme of the Nd ions doped into Y 2 SiO 5 . We use the optical transition at 883 nm between the 4 I 9/2 ground state and 4 F 3/2 excited state. The former is split into two Zeeman levels by a 0.3 T magnetic field (| g 〉 and |aux〉). The experiment is conducted on | g 〉−| e 〉, where the absorption profile is shaped into an AFC by optically pumping atoms into |aux〉. The basic idea is to send in a pulse sequence on | g 〉−| e 〉 that has a periodic spectral density (due its Fourier spectrum). Some of the excited atoms have a certain probability to spontaneously de-excite to |aux〉. The atoms left behind in | g 〉 form the grating (see panel ( b )). To build up a deep grating, the sequence is repeated many times (up to the timescale of the population relaxation between | g 〉 and |aux〉). More details on the preparation can be found in the Experimental setup and Methods section. ( b ) An example of a generated comb with periodicity Δ=10 MHz. The relevant AFC parameters defined in the text are indicated. ( c ) Mapping of weak coherent states with n̄ =0.5 (in a single temporal mode) onto the Nd-doped crystal. Shown are two different experiments with Δ=10 MHz (dashed line offset vertically) and 1 MHz (solid line). The photons that are transmitted without being absorbed are detected at t =0, whereas the absorbed and reemitted photons are detected around t =1/Δ. The vertical scale has been normalized such that it yields efficiency. Inset: The overall write and read efficiency as a function of 1/Δ. Full size image represents one induced optical excitation delocalized over all the N atoms in the comb. In equation (1), z n is the position of atom n , k is the wave number of the single-mode light field, δ n is the detuning of the atom with respect to light frequency and the amplitude c n depends on the frequency and spatial position of the particular atom n . The initial (at t =0) collective strong coupling between the light mode and atoms is rapidly lost because of inhomogeneous dephasing caused by exp( i 2π δ n t ) phase factors. If we assume that the peaks are narrow compared with the periodicity (that is, a high comb finesse F =Δ/ γ ), then δ n ≈ m n Δ (where m n is an integer) and the W state will rephase after a preprogrammed time T =1/Δ. The rephased collective state W will cause a strong emission in the forward direction (as defined by the absorbed light). This type of photon-echo emission is also observed in accumulated or spectrally programmed photon echoes [32] , [33] , [34] , [35] , which inspired our proposal. Spectral atomic gratings have also been proposed [36] and shown [37] for coherent optical delay of streams of strong classical pulses. The interest in spectral gratings was recently renewed in the context of quantum memories, when it was realized how to achieve a much more efficient spectral grating than previously possible. In fact, a 100% efficient echo process is theoretically possible in a backward emission configuration [21] . This is possible because of the highly absorbing and sharp peaks in the AFC structure. In practice, the finite finesse of the comb still needs to be accounted for, which causes a partial loss of the collective state. However, in ref. 21 we show theoretically that F =10 induces a negligible loss, which in combination with a high optical depth d makes the AFC scheme very efficient. High-efficiency mapping using high-finesse combs have recently been shown experimentally [28] , [30] , [31] . These experiments and the present study store light for a predetermined time given by 1/Δ. We thus emphasize that we also proposed [21] and experimentally showed [29] a way to achieve on-demand readout by combining AFC with spin-wave storage. On-demand readout is a crucial resource for applications in quantum networks to render different quantum channels independent. The multimode property of an AFC memory can easily be understood qualitatively. For a periodicity Δ and N p peaks, its total bandwidth is of the order of ∼ N p Δ, indicating that a pulse of duration τ ∼ 1/( N p Δ) can be stored. The multimode capacity stems from the fact that the grating can absorb a train of weak pulses before the first pulse is reemitted after T =1/Δ (see Fig. 1c ). This simple calculation results in a multimode capacity N m ∝ T / τ ∝ N p . Thus, a comb with many peaks, N p , allows us to create a highly multimode memory in the temporal domain. In this context, RE-doped solids are particularly interesting because of their high spectral channel density. Experiment In this study, we work with a neodymium-doped Y 2 SiO 5 crystal, cooled to 3 K, having a transition wavelength at 883 nm with good coherence properties (see Methods for spectroscopic information). This wavelength is convenient as we can work with a diode laser and silicon-based single-photon counters having low noise (300 Hz) and high efficiency (32%). The comb is prepared on the | g 〉−| e 〉 transition by frequency-selective pumping of atoms into an auxiliary state |aux〉 (see Fig. 1 ). There are different techniques for achieving this. For instance, by creating a large spectral hole and then transferring back atoms from an auxiliary state to create a comb, as used in ref. 29 . Here, we use a technique similar to that employed in ref. 22 , in which a series of pulses separated by a time, T , pump atoms from | g 〉 to |aux〉 (through | e 〉) with a power spectrum having a periodicity 1/ T =Δ. This technique is also frequently used in accumulated photon-echo techniques [32] , [37] . Here, each pulse sequence consisted of three pulses in which the central pulse is π-dephased (see Fig. 3c ). This sequence has a power spectrum with 'holes'. A Fourier analysis shows that the width of the holes in the power spectrum decreases when the number of pulses in the sequence increases, resulting in a higher comb finesse. In this experiment, three pulses were enough to reach the optimal comb finesse ( F ≈3) to achieve the maximal efficiency for our optical depth. We refer to the Methods section for more details on the preparation sequence. Figure 3: Increasing spectral bandwidth. 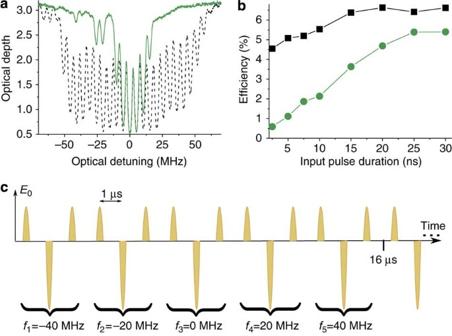Figure 3: Increasing spectral bandwidth. (a) Experimental combs created using preparation sequences with either single (solid line) or five (dashed line) simultaneous pump frequencies. The frequency-shifted sequences allow us to enlarge the frequency range over which the optical pumping is efficient, thereby creating a wide 100 MHz comb. (b) Efficiency as a function of the duration (full-width at half-maximum, FWHM) of the input pulse for a single- (circles) and five (squares)-frequency preparation. As the duration decreases, the bandwidth of the input pulse increases. The decrease in efficiency for short pulses is due to bandwidth mismatch for large bandwidths when using a single-preparation frequency. This experiment clearly illustrates the gain in bandwidth in the extended preparation sequence for which only a small decrease in efficiency is observed. (c) Pulse sequence for atomic frequency comb preparation (see text). To increase the bandwidth, pulses are repeated with shifted frequenciesf=0, ±20 and ±40 MHz. This pulse sequence was used for most of our experiments. Here, it creates a comb of 100 MHz bandwidth and a periodicity of 1 MHz. The total sequence takes 16 μs. ( a ) Experimental combs created using preparation sequences with either single (solid line) or five (dashed line) simultaneous pump frequencies. The frequency-shifted sequences allow us to enlarge the frequency range over which the optical pumping is efficient, thereby creating a wide 100 MHz comb. ( b ) Efficiency as a function of the duration (full-width at half-maximum, FWHM) of the input pulse for a single- (circles) and five (squares)-frequency preparation. As the duration decreases, the bandwidth of the input pulse increases. The decrease in efficiency for short pulses is due to bandwidth mismatch for large bandwidths when using a single-preparation frequency. This experiment clearly illustrates the gain in bandwidth in the extended preparation sequence for which only a small decrease in efficiency is observed. ( c ) Pulse sequence for atomic frequency comb preparation (see text). To increase the bandwidth, pulses are repeated with shifted frequencies f =0, ±20 and ±40 MHz. This pulse sequence was used for most of our experiments. Here, it creates a comb of 100 MHz bandwidth and a periodicity of 1 MHz. The total sequence takes 16 μs. Full size image The experimental sequence is divided into two parts: the preparation of AFC and the storage of weak pulses. To increase the efficiency of optical pumping during the preparation, and thus the depth of the comb, the pulse sequence was repeated 2,000 times, with a delay of 16 μs between each sequence. This is followed by a delay of 5 ms (≈17 T 1 ) to avoid fluorescence noise from atoms left in the excited state. During the storage sequence, 1,000 independent trials are performed at a repetition rate of 200 kHz. The entire preparation and storage sequence is then repeated with a rate of 5 Hz. An overview of the experimental setup is given in Fig. 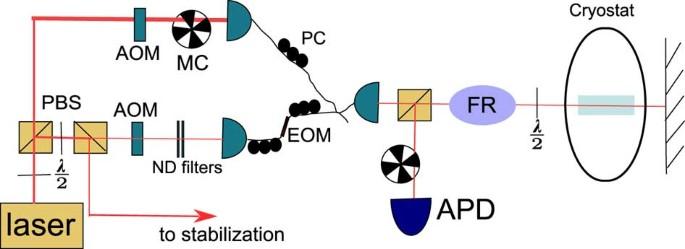2 . Figure 2: Experimental setup. Description of the optical setup used for multiqubit storage experiments. Indicated are the polarization beam splitter (PBS), λ/2 plates, polarization controllers (PC), Faraday rotator (FR), double-pass acousto-optic modulators (AOM), the fast electro-optic amplitude modulator (EOM), neutral density (ND) filters, mechanical choppers (MC) and the silicon single-photon counter (APD). See Methods for more details. Figure 2: Experimental setup. Description of the optical setup used for multiqubit storage experiments. Indicated are the polarization beam splitter (PBS), λ/2 plates, polarization controllers (PC), Faraday rotator (FR), double-pass acousto-optic modulators (AOM), the fast electro-optic amplitude modulator (EOM), neutral density (ND) filters, mechanical choppers (MC) and the silicon single-photon counter (APD). See Methods for more details. Full size image In Fig. 1c, we show storage experiments with predetermined storage times of T =100 ns and 1 μs, for a single temporal mode. The overall in–out mapping efficiencies, defined as the ratio of the output pulse counts to the input pulse counts, are ∼ 6 and ∼ 1%, respectively (see inset of Fig. 1c ). In the Methods section, we present a theoretical analysis of the efficiency performance. The efficiency for single-mode storage is currently lower than that achieved in best-performance single-mode memories, for example, those given in refs [13] , [16] , [17] , [20] , [28] , [30] , [38] 13, 16, 17, 20, 28, 30, 38. However, as explained later, our interface compares very favourably with these experiments in terms of potential multimode storage efficiency. Multimode storage results The main goal of this study is to show high multimode storage. Following the discussion above, we should maximize the number of peaks in the comb. This can be carried out by increasing the density of peaks in a given spectral region (that is, increasing the storage time T ) or by changing the width of the AFC (that is, increasing the bandwidth). Here, we fix the storage time to T =1.3 μs, by which we reach an efficiency of ≳ 1%, and concentrate our efforts on increasing the bandwidth. The spectral width of the grating is essentially given by the width of the power spectrum of the preparation sequence, which, using the pulse sequence described above, only results in a width of about 20–30 MHz. We can, however, substantially increase the total width by inserting more pulses in the preparation sequence, which are shifted in frequency (see Fig. 3c ). We thus optically pump atoms over a much larger frequency range. Note that the frequency shift should be a multiple of Δ to form a grating without discontinuities. In this way, we managed to extend the bandwidth of the interface to 100 MHz, as shown in Fig. 3a , without significantly affecting the AFC echo efficiency. This is illustrated in Fig. 3b , in which we show storage efficiency as a function of the duration of the input pulse when the preparation sequence contains a single or five frequencies. The maximum bandwidth allows us to map short, ≲ 5 ns pulses into memory. In addition to the present motivation for multimode storage, a large bandwidth is equally interesting for interfacing a memory with non-classical single-photon or photon-pair sources. These usually have a large intrinsic bandwidth that requires extensive filtering for matching bandwidths. In this case, our extended bandwidth (×5) would require a corresponding factor of less filtering. We show the high multimode capacity of our interface by storing 64 temporal modes during a predetermined time of 1.3 μs (see Fig. 4 ), with an overall efficiency of 1.3%. This capacity is more than an order of magnitude higher than that previously achieved for multiplexing a quantum memory in a single spatial mode [16] , [22] . As shown, we can store a random sequence of weak coherent states. Storage of random trains of single-photon states has been proposed for multiplexing long-distance quantum communication systems on the basis of the so-called quantum repeaters [5] , [6] . The maximum rate of communication would then be proportional to the number of modes that can be stored [7] . Our experiment clearly shows the gain that can be made using an AFC-based quantum memory. It thus opens up a route towards achieving efficient quantum communication using quantum repeaters. 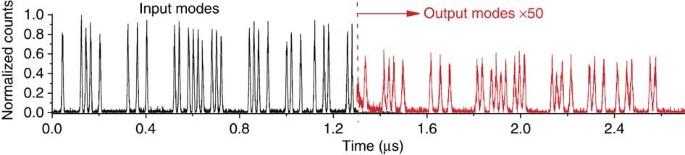Figure 4: Storage of 64 temporal modes. The input (left part) is a random sequence of full and empty time bins, in which the mean photon number in the full ones isn̄≲1. The output (right part) clearly preserves the amplitude information to an excellent degree. The predetermined storage time wasT=1.32 μs; the duration of the input, 1.28 μs; the mode separation, 20 ns; and the mode duration (full-width at half-maximum, FWHM), 5 ns. The output has been multiplied with a factor of 50 for clarity. The average storage and retrieval efficiency was 1.3%. Other examples of multimode storage, for example, with all time bins filled, can be found in theSupplementary Information. Figure 4: Storage of 64 temporal modes. The input (left part) is a random sequence of full and empty time bins, in which the mean photon number in the full ones is n̄ ≲ 1. The output (right part) clearly preserves the amplitude information to an excellent degree. The predetermined storage time was T =1.32 μs; the duration of the input, 1.28 μs; the mode separation, 20 ns; and the mode duration (full-width at half-maximum, FWHM), 5 ns. The output has been multiplied with a factor of 50 for clarity. The average storage and retrieval efficiency was 1.3%. Other examples of multimode storage, for example, with all time bins filled, can be found in the Supplementary Information . Full size image It is now possible to use consecutive temporal modes | k 〉 and | k +1〉 to encode time-bin qubits in which case, a good coherence between modes is crucial. The coherence can be measured by preparing superposition states and performing projective measurements using an interferometric setup. Projective measurements on time-bin qubits are usually performed using an imbalanced Mach–Zehnder interferometer, in which consecutive time bins interfere [1] . We can perform the same task with our light–matter interface using a double-AFC scheme (with Δ 1 and Δ 2 ) as shown in ref. 22 . In short, the difference in delay 1/Δ 1 −1/Δ 2 is the delay in an imbalanced Mach–Zehnder interferometer. The technique used for preparing a double-AFC structure is explained in Methods. As shown in Fig. 5, we observe excellent coherence over all modes with an average visibility of V =86±3%, corresponding to a conditional qubit fidelity of F =(1+ V )/2≈93%. 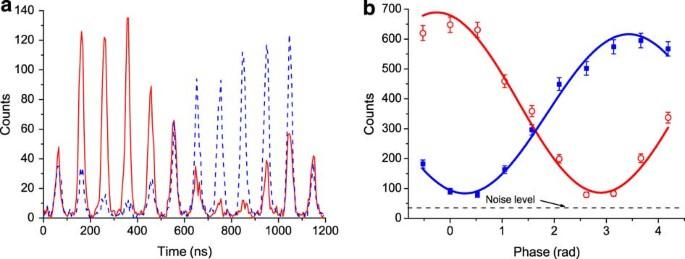Figure 5: Multimode coherence measurement. (a) The output signal (solid line) generated by the double-AFC scheme, which causes an interference between consecutive modes. The input sequence (not shown) is a series of weak coherent states (n̄≈1.8) of equal amplitudeck2, in which the relative phase difference between consecutive modesφk+1−φkranges from −π/6 to 8π/6 with a step of π/6. This allows us to capture a complete interference fringe in one measurement. It also clearly shows the preservation of coherence over the complete multimode output. By changing the detuning of the centre of the second AFC with respect to the carrier frequency of the light, we can impose an additional relative π-phase21on the corresponding output (see Methods). This shifts the interference fringe with half a period (dashed line). (b) The corresponding net interference visibilities are 86±3% (open circles) and 85±3% (filled squares), with detector noise (dashed line) subtracted. The uncorrected raw visibilities were 78±3% and 76±2%. Error bars represent statistical uncertainties of photon counts (±1 s.d.). Figure 5: Multimode coherence measurement. ( a ) The output signal (solid line) generated by the double-AFC scheme, which causes an interference between consecutive modes. The input sequence (not shown) is a series of weak coherent states ( n̄ ≈1.8) of equal amplitude c k 2 , in which the relative phase difference between consecutive modes φ k +1 − φ k ranges from −π/6 to 8π/6 with a step of π/6. This allows us to capture a complete interference fringe in one measurement. It also clearly shows the preservation of coherence over the complete multimode output. By changing the detuning of the centre of the second AFC with respect to the carrier frequency of the light, we can impose an additional relative π-phase [21] on the corresponding output (see Methods). This shifts the interference fringe with half a period (dashed line). ( b ) The corresponding net interference visibilities are 86±3% (open circles) and 85±3% (filled squares), with detector noise (dashed line) subtracted. The uncorrected raw visibilities were 78±3% and 76±2%. Error bars represent statistical uncertainties of photon counts (±1 s.d.). Full size image To further illustrate our ability to store multimode light states, we create a light pulse with a random amplitude modulation. As shown in Fig. 6, we can faithfully store this kind of light pulse. The possibility of storing weak arbitrary light states using photon-echo-based schemes was pointed out already by Kraus et al . (ref. ). We believe that this work, in which complex phase and amplitude information are reversible and coherently mapped onto one atomic ensemble, is the first experimental realization showing these properties at the single-photon level. 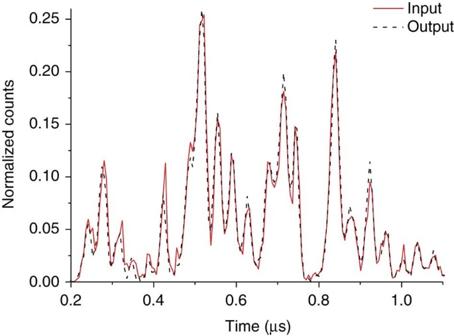Figure 6: Mapping of a randomly amplitude-modulated pulse. As seen, the overlap between the normalized input (dashed line) and output (solid line) pulses is excellent. The total average number of photons in the 1 μs long input pulse isn̄≈4. Figure 6: Mapping of a randomly amplitude-modulated pulse. As seen, the overlap between the normalized input (dashed line) and output (solid line) pulses is excellent. The total average number of photons in the 1 μs long input pulse is n̄ ≈4. Full size image For temporal multimode storage, the efficiency of our interface would outperform the current EIT and Raman-based quantum memories in homogeneously broadened media, although impressive efficiencies have been achieved for single-mode storage [13] , [23] . This is because of the poor scaling of efficiency as a function of the number of modes for a given optical depth [27] . It would also compare favourably with the recent few modes storage experiment [16] using gradient echo memory, another echo-based storage scheme, also because of the scaling of mode capacity for a given optical depth ( N m ∼ d ) [7] , [27] . Nevertheless, an increase in storage efficiency and on-demand readout are necessary for applications in quantum communication. The next grand challenge is to combine multimode storage, high efficiency [30] and on-demand readout [29] in one experiment. The immediate efforts will most probably be devoted to praseodymium- and europium-doped Y 2 SiO 5 crystals, in which the crystal-field ground state has the necessary number of spin levels (three levels) for implementing the on-demand readout. The recent achievements in praseodymium-doped Y 2 SiO 5 crystals are very encouraging [29] , [30] , although the bandwidth was limited to a few MHz because of the hyperfine level splitting. Europium-doped Y 2 SiO 5 has the potential of offering higher bandwidths (up to 70 MHz) and narrower comb peaks, which result in a higher multimode capacity [21] . To exploit the high-bandwidth results reported in this work, using neodymium-doped crystals, one needs to find a third spin level with a long spin coherence lifetime. An interesting path forward is to investigate neodymium isotopes with a hyperfine structure ( 143 Nd and 145 Nd) [39] . Recent results on a similar system [40] , 167 Er 3+ :CaWO 4 , show coherence times approaching 100 μs for hyperfine transitions. Clearly, this path requires extensive spectroscopic studies to optimize the spin population and coherence lifetimes. However, it is very interesting, as it opens up several material candidates (for example, doped with erbium [41] and neodymium) for quantum memory applications. To summarize, we have shown the reversible mapping of up to 64 optical temporal modes at the single-photon level onto one solid-state atomic ensemble. We have shown that the quantum coherence of the stored modes is preserved to a high extent. The different modes can then be used to encode multiple time-bin photonic qubits. Alternatively, they could also be considered as high-dimensional qudit states. This opens up possibilities to store higher dimensional quantum states such as entangled qudits encoded in time-bin bases [42] . Our experiment opens the way to multiqubit quantum memories, which are a crucial requirement for realistic quantum networks. Sample The sample is a 10 mm-long neodymium-doped yttrium orthosilicate crystal (Nd 3+ :Y 2 SiO 5 ) with a low Nd 3+ concentration of 30 p.p.m. The inhomogeneous broadening of the 4 I 9/2 – 4 F 3/2 absorption line is around 6 GHz and the optical depth is 1.5 for this sample (in single-pass configuration), when the polarization of the light is along the D 1 crystallographic axis. We measured an excited state lifetime of T 1 =300 μs using fluorescence spectroscopy and stimulated photon echoes. With conventional photon echoes (two-pulse), we measured a homogeneous linewidth of 3.5 kHz (T 2 =90 μs) for a magnetic field of 300 mT and temperature of 3 K. Each level is a Kramer's doublet that splits into two spin states in a magnetic field. For the field orientation (at 30° relative to the D 2 axis) used in this experiment, we measured g -factors of g g =2.6 and g e =0.5. In a 300 mT magnetic field, the ground and excited states were thus separated by 10.9 and 2.1 GHz. We measured a ground state Zeeman population relaxation lifetime of around T 1 Z =100 ms by spectral hole burning. In the spectral hole-burning measurements, we also observed a superhyperfine interaction of neodymium ions with yttrium. This causes additional spectral side holes at around 640 kHz (for the present magnetic field), thus the effective homogeneous linewidth is around 1 MHz. This was our main limitation for the efficiency of our light–matter interface, as it affected our ability to create a good comb for longer storage times (1/Δ≈1 μs). Experimental setup We present more details on the optical setup shown in Fig. 2 . We used a diode laser that is actively frequency stabilized (<100 kHz), using a spectral hole as reference. The output was split into two beams using a polarization beam splitter. Each beam could be amplitude, frequency and phase modulated using double-pass acousto-optic modulators. One beam was used for creating preparation pulses and the other one for creating the weak pulses to be stored (strongly attenuated using neutral density filters). In the weak path, an additional electro-optic amplitude modulator was used to create short-input pulses for the multimode storage experiments. The paths were mode overlapped using a fibre-coupled beam combiner. The light was sent through the crystal, again in free space, in a double-pass setup to double the optical depth to d =3. Using a Faraday rotator and a λ/2 plate before the crystal, we could separate the input and output modes on the polarization beam splitter, while keeping a constant linear polarization optimized for maximum absorption in the crystal. Output light was collected with a multimode fibre and detected by a silicon single-photon counter. Two synchronized mechanical choppers blocked the detector during the preparation sequence and blocked the preparation beam during the storage sequence. The transmission between the input of the cryostat and the detector was typically between 25 and 30%. Comb preparation We now explain in more detail the preparation sequence allowing us to create the desired comb. The goal is to optically pump atoms from | g 〉 to |aux〉 in a frequency-selective manner (see Fig. 1a ), wherein the atoms left in | g 〉 will form the comb. This can be achieved by two pulses of duration τ separated by time T , as done in ref. [22] 22, which has a power spectrum of width ∼ 1/ τ with a sinusoidal modulation of periodicity 1/ T . To create a sharper comb structure having higher finesse, it is useful to have a wide power spectrum with sharp 'holes' instead of the sinusoidal modulation above. This can be achieved by increasing the number of pulses in the sequence in which the central pulse is π-dephased and has a field amplitude corresponding to the sum of the amplitudes of the side pulses (see Fig. 3c ). In frequency space, the short and intense central pulse interferes destructively with the periodic spectrum of the side pulses, creating a wide power spectrum with the desired holes. From this simple Fourier argument, it is clear that the width of these holes in the spectrum is proportional to the number of pulses. In our study, the optimal finesse is close to 3 for the optical depth of our material, in which case, three pulses were enough to achieve this finesse. For the interference experiment, shown in Fig. 5 , one temporal input mode must be split into two possible temporal output modes. For this purpose, we can create two superimposed combs, with a different periodicity Δ i . An incoming photon then has an equal probability of being absorbed by either of the combs and will consequently be reemitted as a coherent superposition of the two corresponding output modes. To create two combs with periodicity Δ 1 and Δ 2 , we use the sequence shown in Supplementary Fig. S3 . A sequence with N =3 pulses separated by τ 1 is superposed with another sequence of N =3 pulses separated by τ 2 , with the central pulse of each sequence being centred at t =0. Thus, the total number of pulses will be 2 N −1=5, and the pulse area of the central one should be equal to the sum of the others in order to achieve the appropriate interference effect in the power spectrum. It is also possible to impose a phase change φ on the output mode related to a particular comb. This is achieved by frequency shifting the corresponding comb by a fraction of the comb spacing Δ, as discussed in ref. 21 . To do so using our preparation method, we must add a phase to each pulse preparing the corresponding comb (see Supplementary Fig. S3 ). If we label the pulses with k =±1, ±2, ±3… (excluding the central pulse), then the phase of each pulse should be kφ . It is straightforward to show by Fourier analysis that the corresponding power spectrum will see a frequency shift in the position of the holes, which in turn will cause a shift in the position of the created comb. Storage efficiency analysis Efficiency can be calculated theoretically using the formula [21] , [22] . The different terms can be given a qualitative understanding. The first term represents collective coupling, the second the reabsorption of the reemitted light, the third is an intrinsic dephasing factor due to finesse and the last term is a loss due to an absorption background d 0 . For the comb with Δ=10 MHz, we measure d ≈1.7, F ≈2.7 and d 0 ≈0.5 (see Fig. 1b ), resulting in a theoretical efficiency of η ≈5% in close agreement with the experiment (see Fig. 1c ). The major limiting factor here is d 0 (caused by an imperfect preparation of the comb) and then the optical depth of the comb d (the finesse being close to optimum for this d , see ref. ). The decrease in efficiency for longer storage time periods (see inset of Fig. 1c ) is principally due to an increase in background absorption d 0 and an accompanying decrease in peak absorption d . This in turn is caused by the effective spectral resolution of 1 MHz in optical pumping, which is a limitation of the present material (see Methods above). Yet, the storage efficiency is between one and two orders of magnitude higher than that which we achieved in the material Nd:YVO 4 [22] , which we attribute to an improvement in optical pumping in this neodymium-doped material. How to cite this article: Usmani, I. et al . Mapping multiple photonic qubits into and out of one solid-state atomic ensemble. Nat. Commun. 1:12 doi: 10.1038/ncomms1010 (2010).